Generic emergence of classical features in quantum Darwinism Quantum Darwinism posits that only specific information about a quantum system that is redundantly proliferated to many parts of its environment becomes accessible and objective, leading to the emergence of classical reality. However, it is not clear under what conditions this mechanism holds true. Here we prove that the emergence of classical features along the lines of quantum Darwinism is a general feature of any quantum dynamics: observers who acquire information indirectly through the environment have effective access at most to classical information about one and the same measurement of the quantum system. Our analysis does not rely on a strict conceptual splitting between a system-of-interest and its environment, and allows one to interpret any system as part of the environment of any other system. Finally, our approach leads to a full operational characterization of quantum discord in terms of local redistribution of correlations. Our best theory of the fundamental laws of physics, quantum mechanics, has counter-intuitive features (for example, the superposition principle, complementarity and non-locality) that are not directly observed in our everyday classical reality. Furthermore, the postulates of quantum mechanics reserve a special treatment to the act of observation, which contrary to its classical counterpart is not a passive act. The following fundamental questions then naturally emerge: through what process does the quantum information contained in a quantum system become classical to an observer? And how come different observers agree on what they see? The issues of the so-called quantum-classical (QC) boundary and of the related measurement problem dominated large part of the discussions of the early days of quantum mechanics. Indeed, the debate between Bohr and Einstein on the meaning and correctness of quantum mechanics often revolved around the level where quantum effects would disappear—ranging from the microscopic system observed, up to the observer himself. From a practical perspective, our ability to manipulate quantum systems preserving their quantum features has made enormous progress in recent years—enough to purportedly lead A. Zeilinger to state that ‘the border between classical and quantum phenomena is just a question of money’ [1] . However, even if we are somewhat pushing the location of the QC border thanks to our increased experimental ability, a fully satisfactory analysis of the quantum-to-classical transition is still lacking. Such an analysis would both deepen our understanding of the world and conceivably lead to improved technological control over quantum features. Substantial progress towards the understanding of the disappearance of quantum features was made through the study of decoherence [3] , [2] , where information is lost to an environment. This typically leads to the selection of persistent pointer states [3] , while superpositions of such pointers states are suppressed. Pointer states—and convex combinations thereof—then become natural candidates for classical states. However, decoherence by itself does not explain how information about the pointer states reaches the observers, and how such information becomes objective, that is, agreed upon by several observers. A possible solution to these questions comes from an intriguing idea termed quantum Darwinism [4] , [5] , [6] , [7] , [8] , [9] , [10] , [11] , [12] , [13] , [14] , [15] , [16] , [17] , [18] , which promotes the environment from passive sink of coherence for a quantum system to the active carrier of information about the system (see Fig. 1 ). In this view, pointer observables correspond to information about a physical system that the environment—the same environment responsible for decoherence—selects and proliferates, allowing potentially many observers to have access to it. 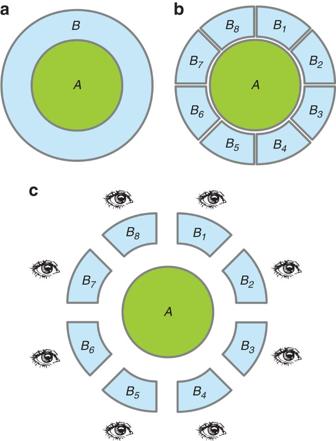Figure 1: Quantum Darwinism treats the environment as carrier of information. (a) The disappearance of quantum coherence in a systemAcan be explained in terms of decoherence induced by the interaction with an environmentB. (b) The environmentBresponsible for decoherence can be thought as being made up of several partsB1,B2,...,Bn. (c) Observers have indirect access to (the information about) systemAthrough their ability to interact with the environment. Each observer is expected to be able to probe only some part of the environment. Only information about the system that is proliferated in the many parts of the environment is effectively available to the observers, and is necessarily classical and objective. Figure 1: Quantum Darwinism treats the environment as carrier of information. ( a ) The disappearance of quantum coherence in a system A can be explained in terms of decoherence induced by the interaction with an environment B . ( b ) The environment B responsible for decoherence can be thought as being made up of several parts B 1 , B 2 ,..., B n . ( c ) Observers have indirect access to (the information about) system A through their ability to interact with the environment. Each observer is expected to be able to probe only some part of the environment. Only information about the system that is proliferated in the many parts of the environment is effectively available to the observers, and is necessarily classical and objective. Full size image The ideas of quantum Darwinism are beautiful and physically appealing. Significant progress was achieved in a sequence of papers [4] , [5] , [6] , [7] , [8] , [9] , [10] , [11] , [12] , [13] , [14] , [15] , [16] , [17] , [18] . However, we are still far from understanding how generally the ideas of quantum Darwinism apply. In particular, for example, given any specific interaction Hamiltonian it is not clear whether and to what extent classicality sets in. A careful and far-from-trivial analysis must in principle be separately performed for each specific model (see the papers cited above). In this paper, we explore whether classical aspects along the quantum Darwinism ideas emerge that are totally independent of the specific dynamics. We prove that some features that are a prerequisite for the validity of quantum Darwinism as explanation for the emergence of classicality are indeed generic. One main consequence of our results is a deep qualitative change in the study of the emergence of classicality: from proving it in given models to showing that it is present in some specific sense in any model involving sufficiently many subsystems of discrete variables. Our results apply beyond the system–environment categorization: in a global system composed of many initially uncorrelated subsystems, any subsystem is being objectively measured by the other ones (see Fig. 2 ). Most importantly, our approach allows to exactly identify which aspects of emergent objectivity are independent from the specific evolution/interaction, and which do instead depend on the model. Indeed the present analysis splits the concept of emergent objectivity into two elements: objectivity of observables and objectivity of outcomes (see Results for detailed definitions). Such two properties ensure that the information about the quantum system does become objective, being accessible simultaneously to many observers and agreed upon. As we report in the Results, the first aspect of objectivity—objectivity of observables—is effectively always present. More specifically, there always exists an explanation for what (most of) the observers see such that they only have at most access to the same classical information about one observable of the system observed. On the other hand, the validity of the objectivity of outcomes depends on how much knowledge about the shared observable is available to the elementary subsystems. Finally, we make use of our techniques to prove in full generality (that is, going well beyond the pure-state case treated in ref. 19 ) that when information is distributed to many parties the minimal average loss in correlations is equal to the quantum discord [20] , a quantity that has recently attracted much attention but was still missing a full clear-cut operational characterization. Our results are related to (and in a sense, an extension of) the no-cloning theorem [21] , and intuitively based on the monogamy of entanglement, as discussed more specifically in Methods. 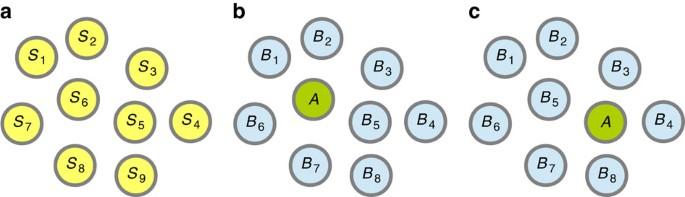Figure 2: Quantum Darwinism beyond the system–environment categorization. (a) We consider the case where we deal with many systemsS1,...,Smthat are initially uncorrelated. (b,c) The role of the system-of-interestAcan be played indifferently by any subsystemSi, with the remaining subsystems playing the role of the (elements of the) environmentB. Thanks to our approach, our results do not depend on any assumed physical symmetry: they are ‘symmetric’ themselves and can be applied for any choice of assignment ‘system-environment’ and any global interaction. We can conclude that any system is being ‘objectively measured’ by the other systems. Figure 2: Quantum Darwinism beyond the system–environment categorization. ( a ) We consider the case where we deal with many systems S 1 ,..., S m that are initially uncorrelated. ( b , c ) The role of the system-of-interest A can be played indifferently by any subsystem S i , with the remaining subsystems playing the role of the (elements of the) environment B . Thanks to our approach, our results do not depend on any assumed physical symmetry: they are ‘symmetric’ themselves and can be applied for any choice of assignment ‘system-environment’ and any global interaction. We can conclude that any system is being ‘objectively measured’ by the other systems. Full size image Physical motivation and notation We want to analyse how the quantum information content of a physical system spreads to (many parts of) its environment. To model this, although our mathematical description in terms of quantum channels (see shortly below) allows for a more general scenario, consider n +1 systems S 1 ,…, S n +1 (see Fig. 2a ). These may constitute a closed system, or be part of a larger system. We focus our attention on one system S i , which we shall call A (see, for example, Fig. 2b ), and we think of the others systems, now denoted B 1 ,…, B n , as of fragments of its environment. All our results assume that A is finite-dimensional, with dimension d A , but we do not need such an assumption for the systems B 1 ,…, B n . Suppose that A is initially decorrelated from B 1 ,…, B n . Independently of any detail of the closed (that is, unitary) or open dynamics of S 1 ,…, S n +1 , this condition ensures that the effective transfer of quantum information from A to B 1 ,…, B n is represented by a quantum channel (also called a quantum operation)—a completely positive trace-preserving (cptp) map— , with the set of density matrices over the Hilbert space X (see Fig. 3 ) [22] . We remark that the role of A can be taken by any S i , as long as it satisfies the condition of being finite-dimensional and initially uncorrelated from the other systems (compare Fig. 2b with Fig. 2c ). 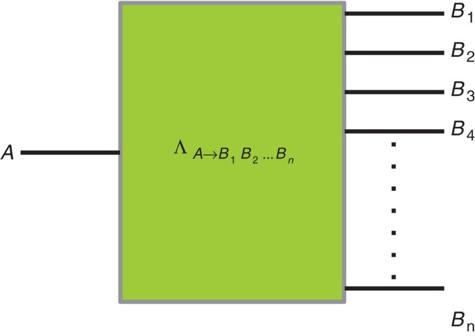Figure 3: The interaction with the environment as quantum channel. The transfer of information from a quantum systemAto the many partsB1B2…Bnof the environment can be described by a quantum channel, that is, a completely positive trace-preserving (cptp) map Λ. Information flows from the left to the right. Figure 3: The interaction with the environment as quantum channel. The transfer of information from a quantum system A to the many parts B 1 B 2 … B n of the environment can be described by a quantum channel, that is, a completely positive trace-preserving (cptp) map Λ. Information flows from the left to the right. Full size image Given two quantum operations Λ 1 and Λ 2 , the diamond norm of their difference is defined as , with the trace norm || X || 1 :=tr(( X † X ) 1/2 ). The diamond norm gives the optimal bias of distinguishing the two operations Λ 1 and Λ 2 by any process allowed by quantum mechanics (that is, choosing the best possible initial state of the system-of-interest and of an ancilla system, applying one of the quantum operations to the first system, and performing the best possible measurement to distinguish the two possibilities) [23] . Thus if , the two maps represent the same physical dynamics, up to error ɛ . Finally, let tr \ X be the partial trace of all subsystems except X . Objectivity of observables and objectivity of outcomes We will adopt the following two notions for emergent objectivity: Objectivity of observables: different observers that access a quantum system by probing part of its environment can only learn information extractable from a single observable of the system (often associated to a measurement on the pointer basis determined by the system–environment interaction [4] ) that, although possibly non-unique, is independent of which part of the environment is being probed. Objectivity of outcomes: different observers that access different parts of the environment have (close to) full access to the information about the above observable and will agree on the outcome obtained ( cf. the agreement condition of ref. 16 ). Our main result about objectivity of observables is as follows (see Fig. 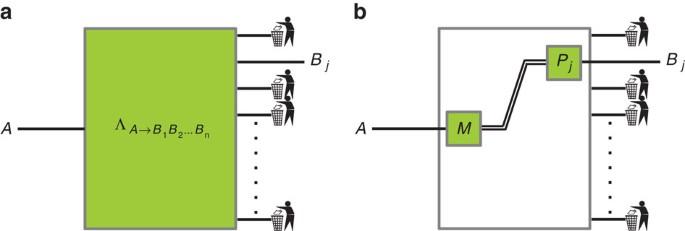Figure 4: The emergence of classicality as due to the distribution of information. (a) The mapping from a systemAto the many partsB1B2…Bnof the environment induces an effective map fromAto each part of the environmentBj, corresponding to tracing out (that is, ‘throwing away’) the rest of the environment. (b) For most of the effective mapsA→Bj, the dynamics can be well-approximated by a measure-and-prepare quantum channel, that is, by a process where the results of a measurementMon the input are used to decide which output to create at a later preparation stagePj. A key point that we prove is that, while the preparation process depends on which partBjof the environment one considers (symbolized by the ‘j’ inPj) the measurement stage is independent of it. This implies that only classical information, and only about a specific measurement onA, is at best accessible to each observer who can only probe a fragmentBjof the environment. Single lines indicate quantum information (qubits); double lines correspond to classical information (bits). Information flows from left to right. 4 ): Figure 4: The emergence of classicality as due to the distribution of information. ( a ) The mapping from a system A to the many parts B 1 B 2 … B n of the environment induces an effective map from A to each part of the environment B j , corresponding to tracing out (that is, ‘throwing away’) the rest of the environment. ( b ) For most of the effective maps A → B j , the dynamics can be well-approximated by a measure-and-prepare quantum channel, that is, by a process where the results of a measurement M on the input are used to decide which output to create at a later preparation stage P j . A key point that we prove is that, while the preparation process depends on which part B j of the environment one considers (symbolized by the ‘ j ’ in P j ) the measurement stage is independent of it. This implies that only classical information, and only about a specific measurement on A , is at best accessible to each observer who can only probe a fragment B j of the environment. Single lines indicate quantum information (qubits); double lines correspond to classical information (bits). Information flows from left to right. Full size image Theorem 1: let be a cptp map. Define as the effective dynamics from and fix a number 1> δ >0. Then there exists a measurement, described by a positive-operator-valued measure (POVM) { M k } k ( M k ≥0, ∑ k M k =I (ref. 22 ), and a set S ⊆ {1,…, n } with | S |≥(1− δ ) n such that for all j ∈ S , with for states . Here d A is the dimension of the space A . As we mentioned before, the diamond-norm distance on the left-hand side of equation (1) represents how different the two physical processes Λ j and are: the smaller the diamond norm, the more similar the processes, to the extent that they can become indistinguishable. The right-hand side of equation (1) is a bound on such a distinguishability that for fixed δ —or even for δ decreasing with n but not too fast, for example, for , for any 0< η <1—becomes smaller and smaller as n increases. So, for fixed d A , in the case where we consider an environment with a large number of parts n (for example, 10 15 ), for all environment parts but δn of them the bound on the right-hand side of equation (1) is very close to zero, that is, the effective dynamics is for all practical purposes. The operation in equation (2) is termed a measure-and-prepare map, since it can be implemented by first measuring the system with the POVM { M k } k and then preparing a state σ j , k depending on the outcome obtained [24] . It is clear that an observer who has access to can at most learn about the measurement of the POVM { M k } k on ρ (but possibly not even that if the states { σ j , k } k are not well-distinguishable). A key aspect of the theorem is that the measurement { M k } k is independent of j . We can interpret { M k } k as the pointer observable of the interaction Λ (see also ref. 18 in this context). In words, the theorem says that the effective dynamics from A to B j , for almost all j ∈ {1,…, n }, is close to a measure-and-prepare channel , with the associated measurement { M k } k the same for all such j . From the perspective of single observers, the evolution Λ is well-approximated by a measurement of A , followed by the distribution of the classical result, which is finally ‘degraded’ by a local encoding that, for each B j , produces a quantum state σ j , k on receiving the result k . Note that the bound is independent of the dimensions of the B subsystems, being therefore very general. Note, however, the dependence on the dimension d A of the system A . Although the functional form of this dependence might be improved, it is clear that no bound independent of d A can exist. Indeed, suppose A = A 1 , …, A n and consider the noiseless channel from A to B 1 ,…, B n , the it is clear that a dimension-independent statement of the theorem would fail. We note that Theorem 1 does not say anything about the second part of quantum Darwinism, namely objectivity of outcomes. It is clear that in full generality this latter feature does not hold true. Indeed, as observed already in ref. 11 , if Λ is a Haar random isometry from A to B 1 ,…, B n , then for any i for which B i has less than half the total size of the environment the effective dynamics from A to B i will be very close to a completely depolarizing one, mapping any state to the maximally mixed state. Therefore objectivity of outcomes must be a consequence of the special type of interactions we have in nature, instead of a consequence of the basic rules of quantum mechanics (in contrast, Theorem 1 shows that objectivity of observables is a consequence only of the structure of quantum mechanics). Can we understand better the conditions under which objectivity of outcomes holds true? First let us present a strengthening of Theorem 1, where we consider subsets of the environment parts. Let [ n ]:={1,…, n }. Theorem 2: Let be a cptp map. For any subset S t ⊆ [ n ] of t elements, define as the effective channel from to . Then for every 1> δ >0, there exists a measurement { M k } k ( M k ≥0, ∑ k M k = I ) such that for more than a (1− δ ) fraction of the subsets S t ⊆ [ n ], with for states . Theorem 2 says that the effective dynamics to B j 1 , . . . B j t is close to a measure-and-prepare channel, for most groups of parts of the environment ( j 1 ,…, j t ). Let us discuss the relevance of this generalization to the objectivity of outcomes question. Let be a block of sites such that the effective dynamics from A to is well-approximated by for the pointer POVM { M k } k and states . From Theorem 2, we know that this will be the case for most of the choices of . As we mentioned before, for many Λ the information about the pointer observable is hidden from any small part of the environment and thus outcome objectivity fails. Suppose, however, that the t observers having access to do have close to full information about the pointer observable. We now argue that this assumption implies objectivity of outcomes. To formalize it, we consider the guessing probability of an ensemble { p i , ρ i } defined by where the maximization is taken over POVMs { N i } i . If the probability of guessing is close to one, then one can with high probability learn the label i by measuring the states ρ i . We have Proposition 3: let be the channel given by equation (5). Suppose that for every i ={1,…, t } and 1> δ >0, Then there exists POVMs such that Equation (7) is equivalent to saying that the information about the pointer observable { M k } k is available to each . Assuming the validity of equation (7), the proposition shows that if observers on measure independently the POVMs , they will with high probability observe the same outcome. Therefore, while objectivity of outcomes generally fails, we see that whenever the dynamics is such that the information about the pointer observable is available to many observers probing different parts of the environment, then they will agree on the outcomes obtained. Deriving quantum discord from natural assumptions Let us now turn to a different consequence of Theorem 1. In the attempt to clarify and quantify how quantum correlations differ from correlations in a classical scenario, Ollivier and Zurek [25] (see also [26] ) defined the discord of a bipartite quantum state ρ AB as where is the mutual information, is the von Neumann entropy, and the maximum is taken over QC channels Γ QC ( X )=∑ k tr( M k X )| k 〉〈 k |, with a POVM { M k } k and orthogonal | k 〉s, which go from the system B to a classical register. These are a special case of the measure-and-prepare channels of equation (2), with the σ states pure and orthogonal. Notice that Ollivier and Zurek originally [25] defined discord in terms of projective measurement rather than general POVMs. The discord quantifies the correlations—as measured by mutual information—between A and B in ρ AB that are inevitably lost if one of the parties (in the definition above, Bob) tries to encode his share of the correlations in a classical system. Alternatively, quantum discord quantifies the minimum amount of correlations lost under local decoherence, possibily after embedding, and in this sense can be linked to the notion of pointer states [25] . As such, quantum discord is often seen as the purely quantum part of correlations, with the part of correlations that can be transferred to a classical system—alternatively, surviving decoherence—deemed the classical part [20] , [25] , [26] , [27] . Recently there has been a burst of activity in the study of quantum discord (see ref. 20 ). Despite the recent efforts, the evidence for a clear-cut role of discord in an operational setting is still limited [20] . Hence it is important to identify situations where discord emerges naturally as the key relevant property of correlations. Here we identify one such setting in the study of the distribution of quantum information to many parties, intimately related to the no-local-broadcasting theorem [27] , [28] . Indeed a corollary of Theorem 1 is the following (see Fig. 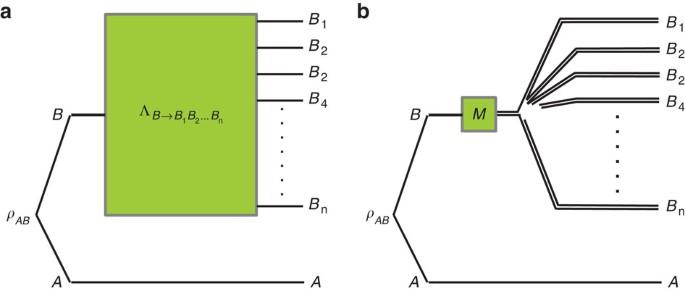Figure 5: Asymptotic distribution of quantum correlations leads to classicality. (a) The partBof a shared stateρABthat contains an amount of correlationsI(A:B)—as measured by mutual informationI—is split and distributed to many partiesB1,B2,...,Bn. We are interested in the largest possible average mutual informationbetweenAand eachBjafter redistribution. That is, roughly speaking, we want to know what is the best possible way to redistribute correlations so that, on average, eachBjis as correlated withAas possible. In a classical scenario this is trivial: everyBjcan be as much correlated withAas the initialB, because it is always possible to broadcast classical information. (b) We find that, as the numbernof recipientsBjgrows the best strategy to redistribute correlations corresponds to reducing it to the classical case in an optimized way. This corresponds to performing the best possible measurement on the original systemB, followed by the distribution of classical information (the outcome of the measurement) to eachBj. Single lines represent quantum information; double lines represent classical information. Information flows from left to right. 5 ; notice that in the following B is a generic system, and so are the systems B 1 , B 2 ,…, B n ): Figure 5: Asymptotic distribution of quantum correlations leads to classicality. ( a ) The part B of a shared state ρ AB that contains an amount of correlations I ( A : B )—as measured by mutual information I —is split and distributed to many parties B 1 , B 2 ,..., B n . We are interested in the largest possible average mutual information between A and each B j after redistribution. That is, roughly speaking, we want to know what is the best possible way to redistribute correlations so that, on average, each B j is as correlated with A as possible. In a classical scenario this is trivial: every B j can be as much correlated with A as the initial B , because it is always possible to broadcast classical information. ( b ) We find that, as the number n of recipients B j grows the best strategy to redistribute correlations corresponds to reducing it to the classical case in an optimized way. This corresponds to performing the best possible measurement on the original system B , followed by the distribution of classical information (the outcome of the measurement) to each B j . Single lines represent quantum information; double lines represent classical information. Information flows from left to right. Full size image Corollary 4: Let be a cptp map. Define ∘ Λ as the effective dynamics from . Then for every 1> δ >0 there exists a set S ⊆ [ n ] with | S |≥(1− δ ) n such that for all j ∈ S and all states ρ AB it holds where , h 2 is the binary entropy function, h 2 ( x )=− x log x −(1− x )log(1− x ), and the maximum on the right-hand side is over QC channels Γ QC ( X )=∑ l tr( N l X )| l 〉〈 l |, with { N l } l a POVM and {| l 〉} l a set of orthogonal states. As a consequence, for every ρ AB , with , and the maximum on the left-hand side taken over any quantum operation . Therefore, we can see the discord of ρ AB as the asymptotic minimum average loss in correlations when one of the parties (Bob, in this case) locally redistributes his share of correlations: Other operational approaches to quantum discord, in particular from a quantum information perspective, have been proposed, but we feel Corollary 4 stands out in comparison to them. First, Corollary 4 does not introduce from the start local measurements, which not so surprisingly would lead to the appearance of discord (as per its definition given in equation (9)); in contrast, measurements appear as ‘effective measurements’ due to the presence of other B ’s. Second, Corollary 4 links quantum discord to the the redistribution of quantum systems and quantum correlations in a general and natural way. Notice that this is different from what done in ref. 29 , where operational interpretations of discord are given that are somewhat more involved, and in ref. 30 , where discord is given an interpretation in quantum communication scenarios that does not really go much beyond its definition. Corollary 4 also has full validity, applying both to the case where ρ AB is a pure state and when it is mixed. In particular this removes the limitations of a recent related work by Streltsov and Zurek [19] . Relation to previous work It is instructive to compare our result to previous work on the subject. In the pioneering works on quantum Darwinism [4] , [5] , [6] , [7] , [8] , [9] , [10] , [11] , [12] , [13] , [14] , the focus was on studying specific examples where the emergence of objectivity could be analysed in detail. We regard Theorem 1 as providing a rigorous justification to some of the claims of those works (namely the basis of the objectivity observables and some aspects of outcome objectivity). The proliferation of information can intuitively be connected to the idea of cloning of information. The no-cloning theorem [21] is one of the hallmarks of quantum mechanics, stating that only classical information can be perfectly and infinitely cloned. Based on this intuition, in two beautiful papers first Chiribella and D’Ariano [31] and later Chiribella [32] obtained the closest results to Theorem 1 previously known (building on refs 33 , 34 ). In those works a variant of Theorem 1 is proven for a dynamics Λ in which all the B subsystems are permutation-symmetric, that is, the information is symmetrically distributed in the environment. In particular, bounds similar to equation (1) were provided, but with the dimension of the B systems in place of the dimension of the A system. Therefore whether the assumption of permutation-symmetry of the B systems (which is to be justified) was needed, and whether the bound had to depend on the dimensions of the outputs (which limits its applicability), were left as open questions until now. Corollary 4 has a similar flavour to a result by Streltsov and Zurek [19] regarding the role of quantum discord in the redistribution of correlations. However, Streltsov and Zurek [19] were only able to treat the case where the initial state shared by Alice and Bob is pure. In such a case it was shown that equation (12) holds even without the need to consider asymptotics, that is, without the limit on the right-hand side of equation (12). We remark that one can take an alternative approach to the study of the validity of the objectivity conditions of quantum Darwinism, not referring at all to the dynamics—as we instead do in this paper—and rather focusing on the properties of the (final) system-environment state. Such an approach was recently considered in ref. 16 by asking what properties the final state of system plus environment should have to satisfy the conditions of ‘objectivity’ in terms of quantum measurement theory. It turns out that from a few assumptions, including Bohr’s non-disturbance principle, full objectivity requires the so-called broadcast structure. The latter has been explicitly shown [17] to be compatible with what a canonical physical model involving photon scattering predicts [12] and with the standard classical information transmission perspective in terms of accessible information [15] (see also ref. 35 for a general perspective). The problem of the quantum-to-classical transition—and in particular, the problem of the origin of classical objectivity—is fascinating. The framework of quantum Darwinism appears as an intriguing possible explanation for it. Quantum Darwinism makes two predictions (which, one could say, constitute its two pillars) on the information about a system that is spread to many observers via the environment that interacts with the system and decoheres it. In this picture, the observers are imagined to acquire information about the system by each having independent access to some part of the environment. The first prediction of quantum Darwinism is objectivity of observables, which states that the environment selects the same specific classical information (that is, information about one specific measurement of the system) to be made potentially available to all the observers. The second prediction is objectivity of outcomes, that is, the fact that the aforementioned observers will (almost) all have access to the outcome of the observation and agree on it. The validity and applicability of the quantum Darwinism approach to the problem of the quantum-to-classical transition were so far only partially understood. The fundamental conclusion of quantum Darwinism theory [4] , [5] , [6] , [7] , [8] , [9] , [10] , [11] , [12] , [13] , [14] , [15] has so far been that the conjunction ‘objectivity of measurements and objectivity of outcomes’ occurs typically in nature because of the specific character of local Hamiltonian interactions. In this work, we have rigorously proven that the first pillar of quantum Darwinism—objectivity of observables—has solid foundations as a consequence of quantum formalism alone (in particular of the monogamy of entanglement [36] , but going beyond the latter). There is always an effective explanation for what the individual observers see that is based on the measurement of one and the same observable (more precisely, one POVM) for (almost) all observers, with the information about the outcome of such observation communicated to each observer in such a way that said information is at most degraded—that is, not fully accessible. Notice that the observers could try to infer information about other observables, but such inference cannot be more successful than trying to infer the value of such observables with processing performed on the quantum signal states that encode the outcome of the measurement of the specified observable. This consideration is in particular relevant for cases where there exist several possibile ‘alternative’ decompositions with the structure of equation (2), and particular some freedom in the identification of the shared observable. Our main result ensures that there is at least one objective observable. This means, on one hand, that, as mentioned, any attempt by the observers at obtaining information about other observables is effectively the same as trying to infer information on such observables from the available information on the one fixed observable. On the other hand, our result—the existence of at least one common observable—is a prerequisite for the selection of a unique observable. The latter uniqueness depends on the properties of the POVM elements M k and of the signal states σ in equation (2), for example, on their (mathematical) linear independence. Thus, while the effective existence of at least a shared observable—from which information about all other observables must be obtained—is independent of the details of the dynamics, its uniqueness does seem to depend on such details. Also the validity of objectivity of outcomes does seem to depend on the details of the interaction, and we are only able to provide partial results about such a feature. Our results seem to indicate that the two pillars of quantum Darwinism are qualitatively different, with the pillar of objectivity of observables a more solid one, because it is deeply rooted in the formalism of quantum mechanics. Our findings suggest that future research should focus on understanding the minimal assumptions needed to ensure the uniqueness of the shared observable and the objectivity of outcomes. Another striking aspect of the generality of our results is that, as mentioned already in the introduction, they actually allow us to go beyond the system–environment categorization. The key point here is that our analysis does not rely on any symmetry assumption about the interaction between the systems S 1 ,…, S n +1 introduced in the first part of the Results section, or about the systems themselves; the conditions of independence and of finite-dimensionality mentioned there suffice to ensure that every system is objectively measured by the others. Up to our knowledge, this is the first result of this generality. A key question is how the present approach can be further generalized to an infinite-dimensional system. This will likely require the consideration of bounds of energy and energy fluctuations, leading to the consideration of an effective dimension for physical systems. Finally, we remark that as a corollary we have also derived a clear-cut operational interpretation to quantum discord, which was originally introduced to capture the quantumness of correlations in information-theoretic terms. We proved that quantum discord corresponds to the asymptotic average loss in mutual information, when one of the parties, for example, Bob, attempts to distribute his share of the correlations with Alice to many parties. From the perspective of quantum Darwinism, one can interpret this result as the fact that the many observers having each access to only a part of the environment will, on average, only be able to establish at most classical correlations with the system-of-interest—the system that ‘gets measured by the environment’. In this sense, we have fully generalized the results of refs 15 , 19 , that were limited to pure states. Proofs The detailed proofs of Theorems 1 and 2, Proposition 3 and Corollary 4 are presented in Supplementary Note 1 , Supplementary Note 2 , Supplementary Note 3 and Supplementary Note 4 , respectively. The proofs rely principally on properties of mutual information that are listed in Supplementary Methods , and make also use of refs 41 , 42 . Here we only provide the proof ideas of Theorem 1, Proposition 3 and Corollary 4. Proof idea of Theorem 1 The proof of Theorem 1 is based on quantum information-theoretic arguments along the lines of recent work by F.G.S.L.B. and Harrow [37] , [38] for deriving new quantum de Finetti theorems. We develop the methods of F.G.S.L.B. and Harrow [37] , [38] further to show that not only the effective channels are close to a measure-and-prepare channel for most j , but that the POVM defining the channels is the same for all j . This latter feature was not appreciated in refs 37 , 38 , but is fundamental in the context of quantum Darwinism. The rough idea of the proof is to consider the state obtained by applying the general dynamics on half of a maximally entangled state of the system A and an ancillary system. This gives the state on AB 1 … B n . Then we consider the effect of measuring (in an appropriate basis that must be optimized over and is not given explicitly) a few of the B j systems of the state , for randomly chosen j ’s. We argue that the statistics of such measurement and the form of the postselected state in system A specifies a POVM { M k } k for which equation (1) holds true. This is a consequence of an important property of the quantum mutual information: the chain rule [22] . Intuitively this process shows that by probing a small part of the environment (with the appropriate measurement) and by considering the effect on the system A , the pointer POVM { M k } k is determined. The argument has connections with the phenomenon of entanglement monogamy [36] , which intuitively says that must be close to a separable state for most j . A state is separable if it can be written as a convex combination of product states: . Thus, by the Choi–Jamiołkowski isomorphism [23] , the associated channel must be close to a measure-and-prepare map. Our results go beyond what we simply expect from entanglement monogamy, by showing the existence of the common pointer POVM for most (which is equivalent to saying that is close to for an ensemble independent of j ). Proof idea of Proposition 3 The proof of Proposition 3 is based on the Gentle Measurement lemma [39] . The latter essentially states that, if a specific outcome of a measurement on a quantum system in a state ρ is highly probable, then, on obtaining that outcome, the state of the system is not changed too much. In the case of the hypotheses of Proposition 3, by distinguishing the single states , an observer can guess with high probability correctly the outcome k . The Gentle Measurement lemma is used to prove that this does not compromise too much the ability of another observer to also obtain the correct result, and hence agree with the first observer. This is generalized to many observers. Proof idea of Corollary 4 The Corollary is based on Theorem 1. The corollary does not use the full power of Theorem 1, as the only important feature in this case is that most of the effective channels to each receiver are close to measure-and-prepare channels. Thus, for a large number of receivers, for most of the latter the amount of correlations with A cannot be greater than the amount of correlations that can be established through a measurement. The additional key property used is the continuity of quantum mutual information, based on the Alicki–Fannes inequality [40] ; this is combined with an opportune scaling of δ with n , so that the averaging over the broadcast receivers makes irrelevant the contribution coming from the (relatively few, that is, sublinear in n ) receivers who potentially have access to a larger amount of correlations. How to cite this article: Brandão, F. G. S. L. et al. Generic emergence of classical features in quantum Darwinism. Nat. Commun. 6:7908 doi: 10.1038/ncomms8908 (2015).